Organizer-derived Bmp2 is required for the formation of a correct Bmp activity gradient during embryonic development Bone morphogenetic proteins (Bmps) control dorsoventral patterning of vertebrate embryos through the establishment of a ventrodorsal gradient of the activated downstream cytoplasmic effectors Smad1/5/8. Some Bmp ligands are expressed in the ventral and lateral regions and in the organizer during gastrulation of the embryo, but it remains unclear how organizer-derived Bmps contribute to total Bmp ligand levels and to the establishment of the correct phospho-Smad1/5/8 gradient along the ventrodorsal axis. Here we demonstrate that interference with organizer-specific Bmp2b signalling in zebrafish embryos alters the phospho-Smad1/5/8 gradient throughout the ventrodorsal axis, elevates the levels of the Bmp antagonist Chordin and dorsalizes the embryos. Moreover, we show that organizer-derived Bmp2b represses chordin transcription in the organizer and contributes to the control of the Chordin gradient. Combining these experimental results with simulations of Bmp’s reaction-diffusion dynamics, our data indicate that organizer-produced Bmp2b is required for the establishment and maintenance of a Bmp activity gradient and for appropriate embryonic dorsoventral patterning during gastrulation. During early embryogenesis, germ layers are induced and patterned in multiple dimensions, and these processes are regulated coordinately by various cellular signals. Some important signalling molecules act as morphogens, forming a concentration or activity gradient to confer specific positional information on embryonic cells at confined locations along the embryonic axes for acquiring a specific fate. The key issues are how a right morphogen gradient is established, maintained and interpreted. Bone morphogenetic proteins (Bmps), ligands of the TGF-β superfamily, are known to function as morphogens during embryonic and organ development [1] , [2] , [3] , [4] . In vertebrate blastulas, Bmp genes are initially ubiquitously expressed and their expression will then cease in the dorsal region while maintain at high levels in the ventral and lateral regions [2] , [4] . In contrast, the Bmp antagonists, primarily Chordin (Chd), are produced in the dorsal organizer region, diffuse ventrally and prevent Bmp ligands from signalling by forming complexes [5] , [6] , [7] , [8] . Bmp ligands usually form heterodimers such as Bmp2/7 or Bmp4/7; the heterodimer binds to and activates the Bmp receptors Alk3/6/8 to phosphorylate the downstream cytoplasmic effectors Smad1, Smad5 or Smad8 that translocate into the nucleus to regulate target gene expression [9] , [10] , [11] . Regional secretion of Bmp ligands and antagonism of Chd in combination with other mechanisms lead to forming of ventral (high) to dorsal (low) activity gradient, that is, the phospho-Smad1/5/8 gradient, which controls embryonic dorsoventral patterning [8] , [12] , [13] , [14] , [15] . Anti-dorsalizing morphogenetic protein (Admp), a Bmp-like protein, is coexpressed with and antagonizes Chd in the organizer by forming Admp/Chd complexes [16] , [17] , [18] , [19] , [20] . Unlike Bmp2/4/7, endogenous Admp may not transduce signal intracellularly, although it can bind to ALK2 in vitro [20] . Knockdown of Admp in frog or zebrafish embryos only causes mild dorsalization [19] , [20] , suggesting that other Bmp members also inhibit Chordin in the organizer. Previous studies have indicated that Bmp genes are transcribed in the organizer field of vertebrate embryos around the onset of gastrulation. In Xenopus , Bmp2 and Bmp7 transcripts are present in the whole marginal zone including the organizer in late blastulas through midgastrulas [21] , [22] , [23] . Zebrafish bmp2b resumes transcription in the embryonic shield (organizer) at the onset of gastrulation [24] , [25] , while bmp4 and bmp7 are transcribed at low levels or not transcribed in the organizer during early gastrulation [13] , [26] , [27] . Mouse Bmp7 transcripts are present in the node, a murine organizer [28] . Therefore, an unsolved issue is whether and how these Bmp transcripts in the organizer contribute to the establishment of the Bmp activity gradient for controlling dorsoventral patterning. In this study, we aimed to elucidate the role of organizer-specific Bmp2b (osBmp2b) in the Bmp activity gradient formation and dorsoventral patterning in the zebrafish embryo. Our experimental data and numerical formulation analysis indicate that osBmp2b is required for establishing and maintaining a correct ventrodorsal Bmp activity gradient to pattern the ventrodorsal axis. Bmp2b is enriched in the organizer of zebrafish embryos A recent study detected endogenous Bmp2b protein in zebrafish embryos by immunofluorescence using an anti-Bmp2b (IN) antibody, but failed to detect Bmp2b in the organizer [13] . We set out to re-investigate Bmp2b distribution using anti-Bmp2b (NT) and anti-Bmp2b (IN) antibodies. In our pilot experiments, we found that immunofluorescence with anti-Bmp2b (NT) produced stronger and clearer signals than an anti-Bmp2b (IN) antibody. The specificity of the anti-Bmp2b (NT) antibody was confirmed in embryos depleted of bmp2b or overexpressing bmp2b mRNA ( Supplementary Fig. 1a–d ). Close-up observation could find some Bmp2b localized to the plasma membrane ( Supplementary Fig. 1e ). These results suggest that this antibody specifically reacts with endogenous Bmp2b. We visualized Bmp2b distribution in embryos by whole-mount immunostaining using anti-Bmp2b (NT) antibody ( Fig. 1e–h ), along with bmp2b mRNA detection by in situ hybridization ( Fig. 1a–d ). We focused on 30–60% epiboly stages since the dorsoventral asymmetry in morphology first appears at the 30% epiboly stage (4.7 h postfertilization (h.p.f. )), gastrulation starts at the 50% epiboly stage (5.3 h.p.f. ), a prominent shield (organizer) is easily visible at the shield stage (6 h.p.f.) and the organizer becomes less distinctive at the 60% epiboly stage (7 h.p.f.) [29] , [30] . From 30 to 50% epiboly stages, Bmp2b formed a ventral (high) to dorsal (low) gradient with the lowest level in the dorsal ( Fig. 1e,f ); by measuring the relative fluorescence intensity (Bmp2b/DAPI) in the ventralmost and dorsalmost areas of equatorial optical sections paralleling the blastodermal margin, a slight increase in the signal along the ventrodorsal axis could be observed ( Supplementary Fig. 2b ). At shield and 60% epiboly stages, the amount of Bmp2b in the ventralmost region was further increased, but an enrichment in the dorsal organizer region was clearly seen ( Fig. 1g,h , and Supplementary Fig. 2b ), which concomitantly occurred with organizer-specific expression of bmp2b mRNA ( Fig. 1c,d ). To verify the existence of osBmp2b, we performed immunofluorescence of cryostat sections of shield stage embryos ( Fig. 1i–p ). Confocal microscopy showed its presence in the organizer region with higher levels in the epidermis ( Fig. 1l,p ). Thus, Bmp2b produced in the organizer may retain locally. Like an anti-Bmp2b (NT) antibody, an anti-Bmp2b (IN) antibody also detected osBmp2b. The failure of osBmp2b detection by Ramel and Hill [13] might be arisen from different experimental procedures. 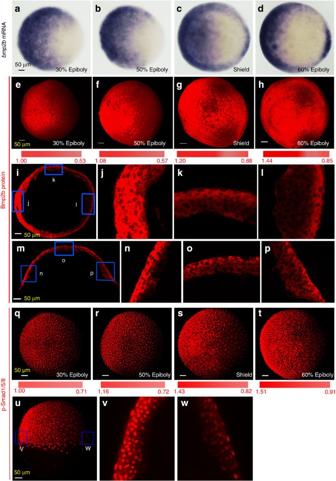Figure 1: Bmp2b mRNA and protein as well as p-Smad1/5/8 are present in the organizer region of zebrafish gastrulas. (a–d) Distribution ofbmp2btranscripts revealed by whole-mountin situhybridization at indicated stages. All embryos were animal-pole views with dorsal to the right. (e–h) Confocal microscopic detection of Bmp2b protein in whole embryos. Embryos at indicated stages were immunostained using an anti-Bmp2b antibody. The z-stack images were shown in animal-pole view with dorsal to the right. The colour bar in (e–h) illustrated signal level changes. The ratio of Bmp2b/DAPI at the two extremes was calculated and indicated. Embryos (3–5), 2–3 sections per embryos, were analysed for each group (also seeSupplementary Fig. 2b, c). (i–p) Confocal microscopic detection of Bmp2b proteins in cryostat sections of embryos at the shield stage. The equatorial (i) or meridional (m) sections, which passed the organizer, were immunostained using an anti-Bmp2b antibody, and the representative z-stack images were orientated with dorsal to the right. The boxed regions in (i) and (m) were enlarged and shown inj–landn–p, respectively. (q–t) Confocal microscopic detection of p-Smad1/5/8. Embryos were immunostained using an anti-p-Smad1/5/8 antibody. The representative z-stack images were shown in animal-pole view with dorsal to the right. (u–w) Distribution of p-Smad1/5/8 in a shield stage embryo. The embryo was laterally viewed with dorsal to the right (u) and boxed ventralmost (v) and dorsalmost (w) areas were enlarged from an optical meridional section. Figure 1: Bmp2b mRNA and protein as well as p-Smad1/5/8 are present in the organizer region of zebrafish gastrulas. ( a – d ) Distribution of bmp2b transcripts revealed by whole-mount in situ hybridization at indicated stages. All embryos were animal-pole views with dorsal to the right. ( e – h ) Confocal microscopic detection of Bmp2b protein in whole embryos. Embryos at indicated stages were immunostained using an anti-Bmp2b antibody. The z-stack images were shown in animal-pole view with dorsal to the right. The colour bar in ( e – h ) illustrated signal level changes. The ratio of Bmp2b/DAPI at the two extremes was calculated and indicated. Embryos (3–5), 2–3 sections per embryos, were analysed for each group (also see Supplementary Fig. 2b, c ). ( i – p ) Confocal microscopic detection of Bmp2b proteins in cryostat sections of embryos at the shield stage. The equatorial ( i ) or meridional ( m ) sections, which passed the organizer, were immunostained using an anti-Bmp2b antibody, and the representative z-stack images were orientated with dorsal to the right. The boxed regions in ( i ) and ( m ) were enlarged and shown in j – l and n – p , respectively. ( q – t ) Confocal microscopic detection of p-Smad1/5/8. Embryos were immunostained using an anti-p-Smad1/5/8 antibody. The representative z-stack images were shown in animal-pole view with dorsal to the right. ( u – w ) Distribution of p-Smad1/5/8 in a shield stage embryo. The embryo was laterally viewed with dorsal to the right ( u ) and boxed ventralmost ( v ) and dorsalmost ( w ) areas were enlarged from an optical meridional section. Full size image The formation and ascent of the Bmp activity gradient Our next question is how dynamic Bmp ligand levels are related to activated downstream effectors. To this end, we visualized p-Smad1/5/8 distribution by immunofluorescence using an anti-Smad1/5/8 antibody. From 30 to 60% epiboly stages, nuclear p-Smad1/5/8 showed a ventral to dorsal gradient with continuous elevation (Fig. 1q–t and Supplementary Fig. 2c ) and did exist in the dorsalmost region ( Fig. 1u–w ). Remarkably, the p-Smad1/5/8 levels in both ventralmost and dorsalmost regions greatly increased after the 50% epiboly stage, and this happened concurrently with the increase of osBmp2b (comparing Fig. 1s,t with Fig. 1g,h ). These observations suggest that (1) Bmp signalling occurs in the dorsal region during early gastrulation; (2) the Bmp activity gradient is initially formed in the late blastula and is further increased and maintained during early gastrulation. osBmp2b contributes to total Bmp2b and p-Smad1/5/8 gradients Since Bmp2b is enriched and is signalling in the organizer, we asked how important osBmp2b signal is for the formation of Bmp2b and p-Smad1/5/8 gradients across the ventrodorsal axis. To tackle these issues, we adopted a strategy to block osBmp2b signalling by overexpressing tBr-gfp transgene driven by a 2.067-kb goosecoid ( gsc ) promoter. As a C-terminally truncated Bmp type I receptor (Alk3), tBr anchored on the membrane is unable to transduce the signal after binding to Bmp2/7 or Bmp4/7 dimers in the extracellular matrix and thereby exhaust free Bmp dimers [31] , [32] , [33] , but it cannot inhibit Admp signalling [17] . Embryos injected with Tg(−2.067gsc:gfp) DNA started to express green fluorescent protein (GFP) weakly around the 30% epiboly stage; at the shield stage, injected embryos (usually >80%) had GFP expression that was restricted to the organizer region ( Supplementary Fig. 3 ). Likewise, embryos injected with Tg(−2.067gsc:tBr-gfp) DNA also displayed a strong GFP expression in the organizer at the shield stage, suggesting an efficient transient expression of tBr-GFP fusion protein ( Supplementary Fig. 3 ). Besides, a 2.272-kb bmp2b promoter could drive the expression of Tg(−2.272bmp2b:gfp) transgene in about 75–85% of injected embryos in the dorsal side at 30–40% epiboly stages and in the organizer at the shield stage ( Supplementary Fig. 4 ), and so this promoter was also used to overexpress tBr-GFP in the organizer. To test effect of tBr overexpression on Bmp2b ligand distribution and Bmp activity gradient, GFP-positive embryos, which were injected with Tg(−2.067gsc:tBr-gfp) or Tg(−2.272bmp2b:tBr-gfp) DNA, were collected at 40% (5 h.p.f.) and 55% epiboly (5.7 h.p.f.) stages and immunostained for Bmp2b and p-Smad1/5/8. Evaluation of relative signal intensity (Bmp2b/DAPI or p-Smad1/5/8/DAPI) at different positions of the equatorial optical sections along the blastodermal margin revealed that tBr-GFP expression driven by either gsc or bmp2b promoter did not cause a significant change of Bmp2b and p-Smad1/5/8 distribution ( Supplementary Fig. 5 ). These observations suggest that Bmp signals in the pre-organizer region before gastrulation, if any, may not be important for the formation of the Bmp2b and p-Smad1/5/8 gradients. Then, we focused on the Bmp2b and Bmp activity distribution at the shield stage following Tg(−2.067gsc:tBr-gfp) injection. Maximal equatorial and meridional cryostat sections passing the organizer were used for immunostaining, and the relative staining intensity in different regions along the ventrodorsal axis was calculated ( Fig. 2 ). Results showed that WT embryos at the shield stage exhibited a V-shape distribution pattern of Bmp2b along the ventrodorsal axis ( Fig. 2a,a′ ), and, in contrast, embryos injected with Tg(−2.067gsc:tBr-gfp) lost this V-shape pattern with a marked decrease throughout the ventrodorsal axis ( Fig. 2b,b′ ). Regarding p-Smad1/5/8, in uninjected embryos at the shield stage, it formed a ventral to dorsal gradient with a much higher intensity in the ventralmost region than in the dorsalmost region ( Fig. 2i–i′′ ); when injected with Tg(−2.067gsc:tBr-gfp) , the gradient was still formed but reduced throughout the ventrodorsal axis ( Fig. 2j–j′′ ). These results suggest that osBmp2b during gastrulation contributes to the establishment and the maintenance of normal Bmp2b and p-Smad1/5/8 distribution along the ventrodorsal axis. 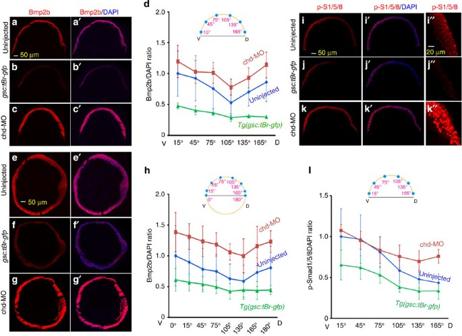Figure 2: Organizer Bmp2b contributes to the formation of correct dorsoventral Bmp2b and p-Smad1/5/8 gradients. (a–d) Changes in Bmp2b protein distribution on meridional sections of differently treated embryos. Meridional cryostat sections passing the organizer of WT (a,a′),Tg(−2,067gsc:tBr-gfp)(b,b′) or chd-MO-injected (c,c′) embryos at the shield stage were immunostained using an anti-Bmp2b antibody along with DAPI staining. The representative confocal images were orientated with dorsal to the right. The average Bmp2b/DAPI signal ratios for indicated ventrodorsal regions of each group of embryos were shown ind. Injection doses (same for others): 105 pgTg(−2,067gsc:tBr-gfp)plasmid DNA; 2.1 ng chd-MO. (e–h) Changes in Bmp2b protein distribution on equatorial sections of differently treated embryos. Equatorial cryostat sections paralleling the blastodermal margin were used for immunostaining. See the above for other necessary information. (i–l) Changes in p-Smad1/5/8 distribution along the ventrodorsal axis in differently treated embryos. Embryos at the shield stage were immunostained using an anti-p-Smad1/5/8 antibody along with DAPI staining. The representative images were optical meridional sections by confocal microscopy with dorsal to the right. The dorsal region ini–kwas enlarged in (i′′–k′′) respectively. The ratios of p-Smad1/5/8 to DAPI signals for indicated ventrodorsal regions of each group of embryos were shown inl. The ratio at each position was averaged from 3 to 5 embryos, 3–5 sections per embryos. The s.d. values were indicated. Figure 2: Organizer Bmp2b contributes to the formation of correct dorsoventral Bmp2b and p-Smad1/5/8 gradients. ( a – d ) Changes in Bmp2b protein distribution on meridional sections of differently treated embryos. Meridional cryostat sections passing the organizer of WT ( a , a′ ), Tg(−2,067gsc:tBr-gfp) ( b , b′ ) or chd-MO-injected ( c , c′ ) embryos at the shield stage were immunostained using an anti-Bmp2b antibody along with DAPI staining. The representative confocal images were orientated with dorsal to the right. The average Bmp2b/DAPI signal ratios for indicated ventrodorsal regions of each group of embryos were shown in d . Injection doses (same for others): 105 pg Tg(−2,067gsc:tBr-gfp) plasmid DNA; 2.1 ng chd-MO. ( e – h ) Changes in Bmp2b protein distribution on equatorial sections of differently treated embryos. Equatorial cryostat sections paralleling the blastodermal margin were used for immunostaining. See the above for other necessary information. ( i – l ) Changes in p-Smad1/5/8 distribution along the ventrodorsal axis in differently treated embryos. Embryos at the shield stage were immunostained using an anti-p-Smad1/5/8 antibody along with DAPI staining. The representative images were optical meridional sections by confocal microscopy with dorsal to the right. The dorsal region in i – k was enlarged in ( i′′ – k′′ ) respectively. The ratios of p-Smad1/5/8 to DAPI signals for indicated ventrodorsal regions of each group of embryos were shown in l . The ratio at each position was averaged from 3 to 5 embryos, 3–5 sections per embryos. The s.d. values were indicated. Full size image Chd downregulates Bmp2b synthesis and p-Smad1/5/8 gradient Chd is believed to inhibit Bmp signalling by associating with Bmp ligands [5] , [34] . However, it is unclear how Chd could affect endogenous Bmp2b protein distribution and consequently Bmp activity gradient. To solve this important question, we knocked down chd expression as reported [35] and examined Bmp2b and p-Smad1/5/8 by immunostaining analysis. We found that the Bmp2b amounts in chd morphants at the shield stage were elevated throughout the ventrodorsal axis so that the V-shape pattern was unchanged ( Fig. 2c,c′ ). Considering that chd knockdown upregulated Bmp2b protein levels at a comparable degree in both dorsal and ventral sides, we hypothesize that Chd, though produced only in a restricted dorsal region, should have a fast diffusion rate to reach and function in the ventral side. Immunostaining of p-Smad1/5/8 detected an increased gradient with a reduced slope in chd morphants at the shield stage ( Fig. 2k–k′′ ). Notably, the p-Smad1/5/8 levels were increased more in the dorsal region, suggesting that repression of Bmp signalling by Chd in the dorsal region is necessary for forming an appropriate Bmp activity gradient. Chd distribution is expanded by exhaustion of osBmp2b The chd gene is specifically transcribed in the dorsal organizer in vertebrate embryos, but it is unknown how its protein product is distributed in late blastulas and early gastrulas because of lack of appropriate antibodies. We found that an anti-Chd antibody (GeneTex) was able to detect endogenous Chd of zebrafish embryos by immunostaining ( Supplementary Fig. 6 ). Then, we investigated the dynamic distribution of Chd in WT embryos. In embryos from 30–60% epiboly stages, the dorsal (high) to ventral (low) gradient of Chd was visible ( Fig. 3e–h , and Supplementary Fig. 2d ); the signal steadily increased in the dorsal region until the shield stage while it was increased a little in the ventral region, which resulted in a steeper gradient ( Supplementary Fig. 2d ). Notably, the Chd protein was distributed well beyond its mRNA distribution area (comparing Fig. 3e–h with Fig. 3a–d ). By focusing the equatorial optical plane at the blastodermal margin of early gastrulas under a higher magnification, we could clearly see the existence of Chd in the ventralmost region in addition to lateral and dorsal regions ( Fig. 3i–k ). Furthermore, Chd was located extracellularly and intracellularly ( Fig. 3l ). Codetection of chd transcripts by in situ hybridization and Chd protein by immunofluorescence in early gastrulas revealed that Chd protein was indeed capable of diffusing far from the Chd-producing cells ( Fig. 3m–p ). This is consistent with non-cell-autonomous action of chd in zebrafish embryos [32] and the ability of endogenous Chd protein to diffuse to the ventralmost side of Xenopus late gastrulas [36] . 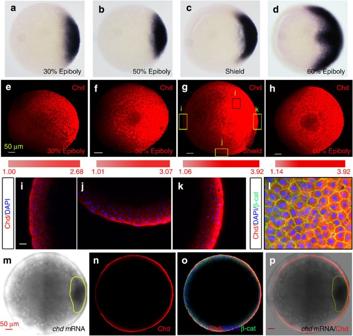Figure 3: Chd protein forms a dorsal to ventral gradient. (a–d)chdmRNA expression detected byin situhybridization in WT embryos at indicated stages. The shown were animal-pole views with dorsal to the right. (e–h) Chd protein distribution in WT embryos at different stages. Embryos were immunostained using an anti-Chd antibody and observed by confocal microscopy. Representative z-stack images were shown with dorsal to the right. The colour bar blow each picture illustrated signal level changes from ventral to dorsal with the ratio of Chd/DAPI at the two extremes indicated (also seeSupplementary Fig. 2d). (i–k) Confocal images of Chd in different regions of embryos at the shield stages. Different regions boxed ingwere viewed in an optical equatorial plane within the blastodermal margin. Note the presence of Chd in the ventralmost region (i). (l) Subcellular localization of Chd in embryos. A region boxed ingwas enlarged. (m–p) Relationship betweenchdmRNA and Chd protein locations in embryos at the shield stage. Embryos were probed with antisensechdRNA probe and then immunostained using anti-Chd and anti-β-catenin antibodies along with DAPI staining. A representative embryo was observed under a confocal microscope in bright field (m) or in fluorescent field (n,o) with a focus plane at the blastodermal margin. Inp, the confocal fluorescence image innwas superimposed on the bright/dark image inm. All images were orientated with dorsal to the right. The border of thechdmRNA area was labelled with a circle. Figure 3: Chd protein forms a dorsal to ventral gradient. ( a – d ) chd mRNA expression detected by in situ hybridization in WT embryos at indicated stages. The shown were animal-pole views with dorsal to the right. ( e – h ) Chd protein distribution in WT embryos at different stages. Embryos were immunostained using an anti-Chd antibody and observed by confocal microscopy. Representative z-stack images were shown with dorsal to the right. The colour bar blow each picture illustrated signal level changes from ventral to dorsal with the ratio of Chd/DAPI at the two extremes indicated (also see Supplementary Fig. 2d ). ( i – k ) Confocal images of Chd in different regions of embryos at the shield stages. Different regions boxed in g were viewed in an optical equatorial plane within the blastodermal margin. Note the presence of Chd in the ventralmost region ( i ). ( l ) Subcellular localization of Chd in embryos. A region boxed in g was enlarged. ( m – p ) Relationship between chd mRNA and Chd protein locations in embryos at the shield stage. Embryos were probed with antisense chd RNA probe and then immunostained using anti-Chd and anti-β-catenin antibodies along with DAPI staining. A representative embryo was observed under a confocal microscope in bright field ( m ) or in fluorescent field ( n , o ) with a focus plane at the blastodermal margin. In p , the confocal fluorescence image in n was superimposed on the bright/dark image in m . All images were orientated with dorsal to the right. The border of the chd mRNA area was labelled with a circle. Full size image We then investigated whether the diffusion of Chd is regulated by osBmp2b signal. We found that, when osBmp2b ligands were inactivated by injection of Tg(−2.067gsc:tBr-gfp) or Tg(−2.272bmp2b:tBr-gfp) DNA, the immunostaining signal level of Chd was not significantly increased by 40 or 55% epiboly stage in either dorsalmost or ventralmost blastodermal margins ( Fig. 4a,b,e,f ); however, Chd intensity appeared increased significantly in both sides at the shield stage ( Fig. 4c,g ). These observations imply that lack of osBmp2b signal promotes production, stability or diffusion of Chd during early gastrulation but not before gastrulation. Thus, osBmp signal can control the Chd gradient after gastrulation starts, which is consistent with the impact of osBmp signal on the Bmp2b distribution and the Bmp activity gradient ( Fig. 2 and Supplementary Fig. 5 ). 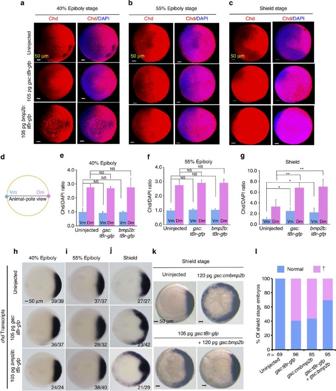Figure 4: Chd protein and transcripts are increased by intervening with organizer Bmp signalling. (a–c) Chd protein distribution detected by confocal microscopy at different stages. Embryos injected withTg(−2.067gsc:tBr-gfp)orTg(−2.272bmp2b:tBr-gfp)DNA were harvested along with uninjected embryos at indicated stages for immunostaining using an anti-Chordin antibody and DAPI staining. Representative z-stack images were shown in animal-pole view with dorsal to the right. (d–g) The average ratios (e–g) of Chd to DAPI signals at the ventralmost or dorsalmost areas on optical equatorial sections at the blastodermal margin as illustrated ind. The strategy for estimating relative intensity was the same as described in the legend ofSupplementary Fig. 2. For each group, the average relative immunostaining intensity was calculated from 3 to 5 embryos and three optical sections at and nearby the blastodermal margin per embryo. The error bars represented s.d. The Chd/DAPI ratio in the ventralmost region at each stage was set to 1.0. Statistical significance (Student’st-test): NS, nonsignificant (P>0.05); *P<0.05; **P<0.01. (h–k)chdtranscripts distribution detected byin situhybridization at indicated stages. Representative embryos were animal-pole views with dorsal to the right. The ratio of embryos with representative pattern was indicated for those shown inh–j(l) The ratio of embryos showing an expansion ofchdexpression at the shield stage (as shown ink)n, number of observed embryos. Figure 4: Chd protein and transcripts are increased by intervening with organizer Bmp signalling. ( a – c ) Chd protein distribution detected by confocal microscopy at different stages. Embryos injected with Tg(−2.067gsc:tBr-gfp) or Tg(−2.272bmp2b:tBr-gfp) DNA were harvested along with uninjected embryos at indicated stages for immunostaining using an anti-Chordin antibody and DAPI staining. Representative z-stack images were shown in animal-pole view with dorsal to the right. ( d – g ) The average ratios ( e – g ) of Chd to DAPI signals at the ventralmost or dorsalmost areas on optical equatorial sections at the blastodermal margin as illustrated in d . The strategy for estimating relative intensity was the same as described in the legend of Supplementary Fig. 2 . For each group, the average relative immunostaining intensity was calculated from 3 to 5 embryos and three optical sections at and nearby the blastodermal margin per embryo. The error bars represented s.d. The Chd/DAPI ratio in the ventralmost region at each stage was set to 1.0. Statistical significance (Student’s t -test): NS, nonsignificant ( P >0.05); * P <0.05; ** P <0.01. ( h – k ) chd transcripts distribution detected by in situ hybridization at indicated stages. Representative embryos were animal-pole views with dorsal to the right. The ratio of embryos with representative pattern was indicated for those shown in h – j ( l ) The ratio of embryos showing an expansion of chd expression at the shield stage (as shown in k ) n , number of observed embryos. Full size image chd transcription is repressed by osBmp2b signalling An interesting question is how osBmp2b controls the Chd gradient. On one way, as evidenced in Xenopus [5] , osBmp2b may form complexes with Chd and promotes Chd degradation by metalloproteases. Another way could rely on transcriptional repression of chd by osBmp2b signalling so that Chd production is limited. To test the second hypothesis, we investigated the regulatory role of Bmp2b in chd transcription. When tBr-GFP was specifically expressed in the organizer by injecting Tg(−2.067gsc:tBr-gfp) or Tg(−2.272bmp2b:tBr-gfp) DNA, embryos showed almost normal chd mRNA expression pattern at 40 and 55% epiboly stages ( Fig. 4h,i ); however, 55–72% of injected embryos at the shield stage displayed a marked expansion of chd expression domain ( Fig. 4j ). The chd expansion caused by Tg(−2.067gsc:tBr-gfp) could be alleviated by coinjection of Tg( −2.067 gsc:bmp2b) plasmid ( Fig. 4k,l ). Overexpression of cmbmp2b in the organizer, which encoded a dominant-negative mutant of Bmp2b that carried 290 RXXR 293 to GVDG mutations in the cleavage site so that mature protein could not be produced [23] (see Supplementary Fig. 7 for its effectiveness), had a similar effect on the chd expression domain ( Fig. 4k ). The expansion of chd transcription area did cohere with the increased amount of Chd protein in embryos on interference with osBmp signalling ( Fig. 4c,g ), suggesting an importance of osBmp signalling in controlling Chd production through transcriptional repression. Thus, the coexpression of Bmp2b and Chd in the organizer provides an important mechanism preventing excess Chd from diffusing to and functioning in the ventral region of embryos. Bmp/Smad signalling directly represses chd transcription We then asked whether Bmp/Smad signalling repressed chd transcription directly or indirectly. To address this question, we isolated a 2,235-bp promoter sequence of the chd locus. The injected transgene Tg(−2.235chd:gfp) was specifically expressed in the dorsal region of gastrulas, which was enhanced by smad5 knockdown ( Fig. 5a ). Another reporter, pGL3( − 2.235chd:luc) , showed a reduced expression level when co-transfected with Smad5 into mammalian Hep3B cells ( Fig. 5b ). These results imply that the isolated chd promoter region contains Bmp/Smad-responsive elements. 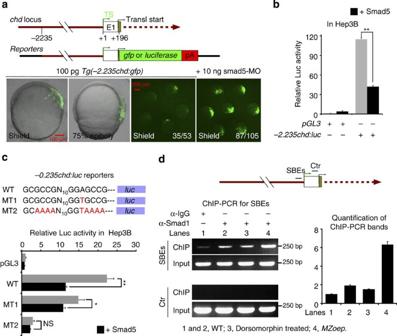Figure 5: Transcription ofchdgene is repressed by Bmp2b signal in the organizer. (a) GFP expression driven by achdpromoter. Top panel illustrated structures of thechdlocus and reporter constructs. TS, transcription start. Bottom panel showedgfpreporter expression in embryos at different stages with the ratio of indicated GFP-positive embryos. (b) Luciferase reporter expression driven by thechdpromoter in Hep3B. ThepGL3(−2.235chd:luc)construct was transfected alone or together with human Smad5, and relative luciferase activity was the mean from three experiments with s.d. indicated. Statistical significance (Student’st-test): **P<0.01. (c) Effect of mutations in definedcis-elements on luciferase reporter expression. The top panel illustrated different constructs and the bottom panel showed luciferase reporter expression in Hep3B cells after transfection with reporter construct alone or together with Smad5. The average with s.d. was calculated from three independent experimental results. Statistical significance (Student’st-test): *P<0.05; **P<0.01; NS,P>0.05. (d) Detection of Smad1 bound tochdpromoter by using ChIP assay. On the top, illustration of the amplified Smad1-occupied region (SBEs) and a control region (Ctr) inchdlocus; left panel in the bottom, ChIP-PCR results; bar graph in the bottom, quantification of the amplified SBEs fragment. The shown were the mean with s.d. from three experiments. Figure 5: Transcription of chd gene is repressed by Bmp2b signal in the organizer. ( a ) GFP expression driven by a chd promoter. Top panel illustrated structures of the chd locus and reporter constructs. TS, transcription start. Bottom panel showed gfp reporter expression in embryos at different stages with the ratio of indicated GFP-positive embryos. ( b ) Luciferase reporter expression driven by the chd promoter in Hep3B. The pGL3(−2.235chd:luc) construct was transfected alone or together with human Smad5, and relative luciferase activity was the mean from three experiments with s.d. indicated. Statistical significance (Student’s t -test): ** P <0.01. ( c ) Effect of mutations in defined cis -elements on luciferase reporter expression. The top panel illustrated different constructs and the bottom panel showed luciferase reporter expression in Hep3B cells after transfection with reporter construct alone or together with Smad5. The average with s.d. was calculated from three independent experimental results. Statistical significance (Student’s t -test): * P <0.05; ** P <0.01; NS, P >0.05. ( d ) Detection of Smad1 bound to chd promoter by using ChIP assay. On the top, illustration of the amplified Smad1-occupied region (SBEs) and a control region (Ctr) in chd locus; left panel in the bottom, ChIP-PCR results; bar graph in the bottom, quantification of the amplified SBEs fragment. The shown were the mean with s.d. from three experiments. Full size image To look for the potential Bmp/Smad-responsive elements, we dissected the 2,235-bp chd promoter by making a series of truncation mutants based on the constructs pGL3( − 2.235chd:luc) and Tg(−2.235chd:gfp) ( Supplementary Fig. 8a ). The reporter assays in mammalian cells and in fish embryos indicated that a 235-bp proximal region was required for response to Smad1/5 stimulations or repression ( Supplementary Fig. 8b–f ). Examination of the 235-bp promoter sequence identified two potential Smad1/5-binding elements, 5′-GCGCCG-3′ and 5′-GGAGCCG-3′ ( Fig. 5c ), belonging to a novel class of Smad1/5-bind motifs [37] . When the distal element was mutated, the luciferase reporter expression in Hep3B cells was reduced but still responsive to Smad5 repression; however, mutations in both elements resulted in a greater reduction of the reporter expression and loss of responsiveness to Smad5 repression ( Fig. 5c ). The effect of these mutations on GFP or luciferase reporter expression was confirmed in zebrafish embryos ( Supplementary Fig. 9 ). Thus, these Smad1/5-binding elements are required for responsiveness to Smad1/5 repression. We next investigated whether the identified elements could be bound by Smad1/5 in zebrafish embryos. Chromatin-immunoprecipitation (ChIP) using an anti-Smad1 antibody indicated that a region spanning those elements was enriched in the precipitated DNAs ( Fig. 5d ). Inhibition of Bmp signalling in embryos by treating with the inhibitor Dorsomorphin slightly reduced the amount of the amplified Smad1-bound sequence ( Fig. 5d ). In MZoep embryos deficient for Nodal signalling [38] , the amount of the Smad1-bound sequence was remarkably increased ( Fig. 5d ), suggesting that Smad2/3 may compete with Smad1/5 for those elements. Therefore, we conclude that activated Smad1/5 in the organizer directly binds to and represses the transcription activity of the chd promoter. osBmp2b is required for embryonic dorsoventral patterning We have demonstrated in the above sections that osBmp2b participates in the formation of a proper ventral to dorsal Bmp activity gradient. A biological question is whether it is required for normal embryonic dorsoventral patterning and development. We blocked osBmp2b signalling by injecting Tg(−2.067gsc:tBr-gfp) , Tg(−2.067gsc:cmbmp2b), Tg(−2.272bmp2b:tBr-gfp) or Tg(−2.272bmp2b:cmbmp2b) DNA at the one-cell stage and found that tBr-GFP or Cmbmp2b expression driven by either promoters led to severe embryonic dorsalization at 24 h.p.f. ( Fig. 6a,b ). In contrast, bmp2b overexpression in the organizer caused embryonic ventralization ( Fig. 6a,b ). Examination of dorsal and ventral markers at the shield stage revealed an increase of the dorsal markers floading head ( flh ) and gsc and a decrease of the ventral maker eve1 when tBr or Cmbmp2b was expressed ( Fig. 5c,d ). The effect of tBr-GFP on these markers expression could be compromised by co-overexpression of Tg(−2.067gsc:bmp2b) ( Supplementary Fig. 10 ), demonstrating a specific effect. Taken together, these results indicate that osBmp2b signalling is necessary for normal dorsoventral development. 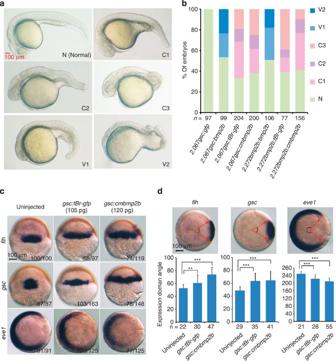Figure 6: Altered organizer Bmp2b signalling levels disrupt embryonic dorsoventral patterning. (a) Representative morphology of different categories of live embryos at 24 h.p.f. after injection. Plasmid DNA was injected at doses: 105 pg forTg(−2.067gsc:gfp),Tg(−2.067gsc:tBr-gfp)andTg(−2.272bmp2b:tBr-gfp); 120 pg for the other constructs. (b) The ratio of embryos in different categories following injection of different plasmids.n, the number of observed embryos. (c) Marker expression detected byin situhybridization at the shield stage. Embryos forflhandgscwere dorsally viewed and those foreve1were viewed from the animal-pole with dorsal to the right. The ratio of embryos with the representative expression pattern was indicated. Amplified transgene DNA fragments from corresponding constructs were used for injection. (d) Quantification of marker expression domains. The angle for each marker, as depicted in the top of each bar graph, was measured and averaged with s.d. indicated (bottom).n, the number of observed embryos. Statistical significance (Student’st-test): **P<0.01; ***P<0.0001. Figure 6: Altered organizer Bmp2b signalling levels disrupt embryonic dorsoventral patterning. ( a ) Representative morphology of different categories of live embryos at 24 h.p.f. after injection. Plasmid DNA was injected at doses: 105 pg for Tg(−2.067gsc:gfp) , Tg(−2.067gsc:tBr-gfp) and Tg(−2.272bmp2b:tBr-gfp) ; 120 pg for the other constructs. ( b ) The ratio of embryos in different categories following injection of different plasmids. n , the number of observed embryos. ( c ) Marker expression detected by in situ hybridization at the shield stage. Embryos for flh and gsc were dorsally viewed and those for eve1 were viewed from the animal-pole with dorsal to the right. The ratio of embryos with the representative expression pattern was indicated. Amplified transgene DNA fragments from corresponding constructs were used for injection. ( d ) Quantification of marker expression domains. The angle for each marker, as depicted in the top of each bar graph, was measured and averaged with s.d. indicated (bottom). n , the number of observed embryos. Statistical significance (Student’s t -test): ** P <0.01; *** P <0.0001. Full size image An interesting question is what would happen to embryos if both organizer Bmp signalling and Chd production are prevented. To this end, we observed morphological changes in 26-h.p.f. embryos following coinjection of Tg(−2.067gsc:tBr-gfp) and chd-MO. We observed that chd-MO-induced embryonic ventralization was aggravated by simultaneous inhibition of organizer Bmp signalling ( Supplementary Fig. 11 ). Thus, in the absence of osBmp and Chd, ventrolateral Bmp activity is sufficient to ventralize embryos. The result also supports the notion that tBr-GFP expressed from Tg(−2.067gsc:tBr-gfp) does not intervene in Bmp signalling outside the organizer. Mathematic modelling of the Bmp activity gradient The reaction-diffusion dynamics of the Bmp morphogen activity gradient has been investigated previously [14] , [39] , [40] , but effect of Bmp2/7 synthesized in the organizer field on this dynamic process has not been taken into account. We tried to develop a theoretical model to show how the reaction-diffusion dynamics of Bmp signals is influenced by osBmp signalling. For simplicity, we mainly focused on biochemical reactions between the Bmp antagonist Chd ( C ) and two sources of Bmp ligands, ventral Bmp ligands (vBmp) ( L ) and osBmp ligands ( L′ ), which can form LC and L′C complexes ( Supplementary Fig. 12 ). We regarded free Bmp ligands as those that were not bound by Chd and could transduce the signal intracellularly. The synthesis of vBmp was assumed to be positively regulated by total free Bmp level as evidenced previously [24] , [41] , [42] , while the synthesis of Chd was assumed to be controlled by a negative feedback function of total free Bmp level in the organizer as shown in Fig. 4 . Like simulations in Xenopus [14] , we considered only one-dimensional geometry in the zebrafish embryo, that is, the ventrodorsal axis. The formulation of the reaction-diffusion dynamics was described in detail in Methods. On the basis of previous models [14] , [39] , [40] , we set the parameters in the numerical simulations ( Supplementary Table 1 ). We simulated the diffusion dynamics of the total Bmp level (=[ L + L′ + LC + L′C ]), the free Bmp level (=[ L + L′ ]) and the Chd level over the time range from sphere (4 h) to shied (6 h) stages, and numerical results were shown in Fig. 7 . In WT embryos, the total Bmp level and the free Bmp level both remain constant on the x -axis (ventrodorsal axis) at time t =4 h ( Fig. 7a,d ), at which Chd synthesis starts in the organizer ( Fig. 7g ). Because of inhibition of Bmp signals by Chd (forming LC complexes), a Bmp ventral (high) to dorsal (low) gradient gradually forms with the increase of time ( Fig. 7a ). On the basis of our experimental data ( Figs 1a,b and 4 and Supplementary Fig. 5 ), we assume that osBmp re-starts to be synthesized at time t =5.7 h (55% epiboly stage), which corresponded to τ L ′ in equation (2) (see Methods). Because the osBmp ligands consume some Chd in the organizer by forming the complex L′C , the free Bmp gradient on the x -axis will evolve to an appropriate level at time t =6 h ( Fig. 7d,j ). In case that no osBmp is synthesized, the total Bmp and free Bmp levels on the whole x -axis will be lower significantly than that in WT embryos at time t =6 h ( Fig. 7b,e,i,j ), which suggests that osBmp is critical for establishing and maintaining appropriate levels of total Bmp ligands and free Bmp gradient. If no Chd is synthesized, the levels of total Bmp and the free Bmp gradient will approach a higher level on the whole x -axis at time t =6 h ( Fig. 7c,f,i,j ), which suggests an important role of Chd in controlling the free Bmp gradient. In addition, in the absence of osBmp, the Chd dorsal to ventral gradient will be evidently increased at time t =6 h ( Fig. 7h,k ), supporting the role of osBmp in controlling Chd synthesis. Although we did not assume a specific Bmp ligand in our numerical simulations, most of these simulation results well match our experimental data including the dynamic changes of Bmp2b, p-Smad1/5/8 and Chd levels along the ventrodorsal axis in WT, tBr-GFP-overexpressing or chd -knockdown embryos. One discrepancy is that, in case of depletion of Chd, the ventral free Bmp level ( Fig. 7j ) is increased more markedly than the p-Smad1/5/8 level ( Fig. 2l ). This phenomenon may be explained that the ventral free Bmp level in WT embryos is sufficient to maximize the activation of Smad1/5/8 and its further increase in the absence of Chd could not lead to activation of more Smad1/5/8 due to other limiting factors. Taken together, our theoretical and experimental data strongly support the idea that osBmp ligands are required in establishing and maintaining an appropriate Bmp activity gradient around the shield stage. 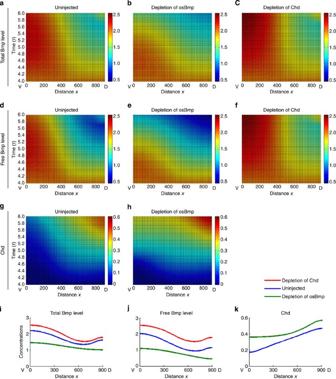Figure 7: Numerically simulated dynamics of total Bmp and free Bmp levels and Chd gradient. Free Bmp ligands represent those unbound by Chd, while total Bmp ligands include free Bmp ligands and Bmp ligands bound to Chd. (a–h) The time dynamics of total Bmp and free Bmp levels and Chd gradient during a specific period of embryonic development. Thex-axis represented the length of the ventrodorsal axis, which was taken in the range 0≤x≤900μm (that is, from the ventral extreme (V) to the dorsal extreme (D)). They-axis denoted the time course being from sphere (4 h) to shield stages (6 h). The colour bar to the right of each picture indicated the concentration levels. Note that Bmp ligands present before the re-start of Bmp synthesis around 5.7 h are presumably remnants synthesized frombmpmRNAs expressed during midblastulation. (i–k) Total and free Bmp levels and Chd gradient at timet=6 h. Figure 7: Numerically simulated dynamics of total Bmp and free Bmp levels and Chd gradient. Free Bmp ligands represent those unbound by Chd, while total Bmp ligands include free Bmp ligands and Bmp ligands bound to Chd. ( a – h ) The time dynamics of total Bmp and free Bmp levels and Chd gradient during a specific period of embryonic development. The x -axis represented the length of the ventrodorsal axis, which was taken in the range 0≤ x ≤900μm (that is, from the ventral extreme (V) to the dorsal extreme (D)). The y -axis denoted the time course being from sphere (4 h) to shield stages (6 h). The colour bar to the right of each picture indicated the concentration levels. Note that Bmp ligands present before the re-start of Bmp synthesis around 5.7 h are presumably remnants synthesized from bmp mRNAs expressed during midblastulation. ( i – k ) Total and free Bmp levels and Chd gradient at time t =6 h. Full size image The Bmp activity morphogen regulates differentiation of cell fates along the ventrodorsal axis during dorsoventral patterning. In vertebrate embryos, an appropriate ventral to dorsal Bmp activity gradient would not be formed in the absence of its antagonist Chd originated from the organizer. Our immunofluorescent assay using an anti-Chd antibody for the first time detected the existence of the dorsal to ventral Chd gradient throughout the zebrafish blastoderm including the ventralmost region from 30 to 60% epiboly stages ( Fig. 3e–h ). When chd is knocked down, the p-Smad1/5/8 level is markedly increased in the dorsal side, whereas the level shows little increase in the ventral side ( Fig. 2k–l ). This observation suggests that inhibition of Bmp signalling by Chd helps form a steep Bmp activity gradient so that cells at different positions along the ventrodorsal axis can receive and respond to distinguishable positional information. In zebrafish, bmp2b mRNA and Bmp2b protein are enriched in the dorsal organizer field immediately after the start of gastrulation (50% epiboly stage) ( Fig. 1a–p ); bmp4 appears weakly expressed and bmp7a is not expressed in that field ( Supplementary Fig. 13 ). Activated Smad1/5/8 is apparently present in the organizer field ( Fig. 1q–w ). We demonstrate that Bmp ligands and their signalling in the organizer field contribute to the establishment of an appropriate ventrodorsal Bmp activity gradient during gastrulation and thereby are necessary for normal dorsoventral patterning. Given the expression of Bmp genes in the organizer/node of Xenopus and mouse [21] , [22] , [23] , [28] , the function of organizer/node Bmp signalling may be conserved across vertebrate species. Coexpression of Bmp2b and Chd in the organizer field should largely allow the formation of Bmp2b/Chd complexes. A question is what the fates of Bmp2b/Chd complexes are. In Drosophila , Dpp/Sog complexes formed in the ventral lateral cells are believed to transport to the dorsal cells in which Sog is cleaved to release Dpp [39] , [43] , [44] . If the same mechanism should be utilized for Bmp2b/Chd complexes in zebrafish embryos, we should see a reduction of Chd distribution range when Bmp2b is exhausted by overexpressed tBr in the organizer. The organizer-specific overexpression of tBr-GFP or Cmbmp2b, which is presumed to reduce the amount of Bmp2b available for binding to Chd due to tBr-GFP/Bmp2b or CmBmp2b/Bmp2b complexes formation, caused ectopic transcription of chd in lateral blastoderm margin but not in the animal-pole area at the shield stage ( Fig. 4j–l ); however, accumulation of Chd protein in the animal-pole area seemed unaffected by exhaustion of osBmp2b ( Fig. 4c ), indicating a long range of diffusion. Therefore, Bmp2b does not promote ventral diffusion of Chd. Given that bmp1- and tll -encoding metalloproteases are expressed in both ventral and dorsal cells of zebrafish embryos [45] , [46] , [47] , Bmp2b/Chd complexes may facilitate Chd degradation in the organizer so that not too much Chd could diffuse to the ventral side (see the model in Supplementary Fig. 14 ). This hypothesis needs to be further investigated in the future. Transcriptional repression of chd by osBmp signalling should be another important mechanism for preventing biosynthesis of excess Chd proteins, helping establish and maintain an appropriate Bmp activity gradient ( Supplementary Fig. 14 ). The previously accepted theories hypothesize that Bmp ligands in the organizer are mainly diffused from the ventral region and are unable to transduce signal due to association with Chd [4] , [15] . We found that Bmp signalling is not fully repressed in the organizer, as evidenced by the increasing amounts of p-Smad1/5/8 in the dorsal side from 30 to 60% epiboly stages ( Fig. 1q–t ). Another important line of evidence is that inhibition of osBmp2b signalling by organizer-specific tBr-GFP overexpression leads to more chd transcripts at the shield stage ( Fig. 4j,k ). Smad1/5/8 can directly bind to the promoter of chd and downregulate its transcription ( Fig. 5a–d ). The amount of p-Smad1/5/8 in the organizer is low compared with the ventral region in normal gastrulas, but can modulate chd transcription there. Probably, some mediators/cofactors in the organizer promote the repression activity of Smad1/5/8. Another interesting phenomenon is that deficiency of osBmp2b signal lowers Bmp2b and p-Smad1/5/8 protein amounts not only in the dorsal but also in the ventral region around the shield stage ( Fig. 2 ). It is well known that Bmp signalling can feed back to activate the expression of Bmp genes in Drosophila , Xenopus and zebrafish embryos [24] , [41] , [42] . We found that inhibition of osBmp2b signalling caused ectopic chd transcription in lateral, even ventral blastoderm margin ( Fig. 4j,k ), which could be ascribed to a decrease of the p-Smad1/5/8 gradient ( Fig. 2j–j′′ ) to the level below the threshold required for efficiently repressing chd transcription in those regions. The increased amount of Chd throughout the embryos ( Fig. 4c,g ) can feed back to block Bmp signalling, ultimately reducing both activated Smad1/5/8 and Bmp2b amounts in the whole embryo. In agreement with this speculation, bmp2b mRNA levels are reduced in ventral and lateral regions in the absence of osBmp signals ( Supplementary Fig. 15 ). The bmp2b mRNA levels appeared unaltered in the organizer of embryos expressing tBr-GFP ( Supplementary Fig. 15 ), but Bmp2b protein level was reduced there ( Fig. 2d,h ). Probably, the formation of Chd/Bmp2b complexes in the organizer accelerates Bmp2b degradation via an unknown mechanism. Nevertheless, controlling of chd transcription by osBmp2b is an important mechanism for the maintenance of the Bmp activity gradient along the ventrodorsal axis during gastrulation. Why is Bmp2b in the organizer required around the shield stage? To understand this, we should take account of the spatiotemporal expression patterns of chd and bmp genes. bmp2b, bmp4 and bmp7 are ubiquitously expressed during midblastula stages, presumably setting up high levels of Bmp ligands in the whole blastoderm [13] . To establish a ventral to dorsal Bmp activity gradient, the embryo around the dome stage (4.3 h.p.f.) seeks a reduction in Bmp activity in the future organizer region (dorsal blastodermal margin) by adopting two strategies: expressing the Bmp antagonist genes such as chd and ceasing bmp2b / bmp4 / bmp7 expression in the dorsal margin. The absence of Bmp ligands in the dorsal margin would allow a fast ventral diffusion of Chd. As the embryo continues developing, more and more Chd proteins are enriched in the dorsal region ( Fig. 3e–h ) and the amount of Chd becomes beyond a demand at the onset of gastrulation. Then, bmp2b is chosen to be re-expressed in the organizer soon after the onset of gastrulation. In addition to repressing chd transcription, osBmp2b may act to buffer the noise in the dorsolateral regions, as demonstrated in other morphogen systems [48] , [49] , [50] , to make the Bmp morphogen stable. Admp is specifically expressed in the dorsal organizer in Xenopus and zebrafish embryos [16] , [18] , [19] . Studies in Xenopus suggest that Admp/Chd complexes formed in the organizer are transported ventrally, so facilitating Chd degradation in the ventral region [14] , [51] , [52] . We found that, when admp was knocked down, the Chd protein distribution was largely unchanged, even though the chd mRNA domain expanded ventrally ( Supplementary Fig. 16 ). Thus, Admp may not act as a carrier of Chd in zebrafish embryos and instead it may regulate dorsoventral patterning through a mechanism different from osBmp2b. Given that Bmp proteins could associate with Nodal in vitro [53] , Admp may antagonize the dorsalizing effect of Nodal proteins. In addition to chd , zebrafish embryos express other Bmp antagonist genes such as nog1 , nog2 , nog3 , fst1 , fstl1 , fst2 and fstl2 . Except nog1 and fstl2 expressing in the organizer, other genes are not expressed during embryonic dorsoventral patterning [54] , [55] , [56] . Loss-of-function of either nog1 or fstl2 does not affect dorsoventral patterning [56] , excluding the possibility of their implication in dorsoventral patterning. Because chd / dino mutant embryos are ventralized [7] , [57] , Chd appears to be a major Bmp antagonist during dorsoventral patterning of zebrafish embryos. In summary, our data indicate that Bmp2b ligands are enriched in the organizer region during early gastrulation in the zebrafish embryo. The production of Bmp2b in the organizer is an effective way to antagonize Chd in the Chd-synthesizing region so that an appropriate Bmp morphogen activity gradient is maintained. Zebrafish strains Tubingen strain of zebrafish was used with ethical approval from the Animal Care and Use Committee of Tsinghua University. Embryos were staged according to Kimmel et al . [30] and specific stages were indicated in the text and figures. MZoep mutant embryos were generated by crossing homozygous male and female oep tz257 mutant fish that were rescued by injecting oep mRNA [38] . Constructs The 2,067-bp promoter of gsc was amplified by PCR from genomic DNA using a pair of specific primers: forward primer, 5′-TTCTTCTGGTCAGTGATTGT-3′ and reverse primer, 5′-ACGAGTGTCCTTCATAGTG-3′. A region containing the 2,235-bp putative promoter of the chd locus was amplified using the forward primer (5′-CCTAACGGTTGAGATTGATAC-3′) and the reverse primer (5′-GATGCGATAATAACGGACAG-3′). The amplified DNA fragments were individually cloned into a pGL3 , a luciferase reporter plasmid (Promega), to generate the corresponding constructs pGL3(−2.067gsc:luc) and pGL3(−2,235chd:luc) for transfection in mammalian cells. The luciferase coding sequence of the above constructs was replaced by the EGFP coding sequence to generate the constructs Tg(−2.067gsc:gfp) and Tg(−2,235chd:gfp) for GFP expression in embryos. The sequence encoding tBr was inserted in frame into the front of gfp of Tg(−2.067gsc:gfp) to make Tg(−2.067gsc:tBr-gfp) . The cmbmp2b coding sequence contains a sequence of 5′-GGCGTTGACGGC-3′ (encoding GVDG) mutated from 5′-CGAGAAAAGCGG-3′ (encoding REKR for propeptide cleavage) of wild-type bmp2b . A 2,620-bp region including a 2,272-bp sequence upstream of bmp2b transcription start site, which contains several Boz-binding sites [58] , and a 348-bp downstream sequence was amplified using the forward primer (5′-CATTGCTCCTCTTCCCAGTT-3′) and the reverse primer (5′-CGTTCCCGTCGTCTCCTAAG-3′) and used for making the construct Tg(−2,272bmp2b:gfp), Tg(−2,272bmp2b:tBr-gfp) , Tg(−2,272bmp2b:bmp2b) and Tg(−2,272bmp2b:cmbmp2b) . mRNAs, morpholinos and microinjection mRNAs were synthesized in vitro from corresponding linearized plasmids using the mMessage mMachine kit (Ambion). The following morpholinos were used: bmp2b-MO, 5′-GTCTGCGTTCCCGTCGTCTCCTAAG-3′ (ref. 59 ); smad1-MO, 5′-AGGAAAAGAGTGAGGTGACATTCAT-3′ (ref. 60 ); smad5-MO, 5′-AACAGACTAGACATGGAGGTCATAG-3′ (ref. 61 ); chd-MO, 5′-ATCCACAGCAGCCCCTCCATCATCC-3′ (ref. 35 ); admp-MO, 5′-TGGACAACATTGTAAAGAACATTGC-3′ (ref. 18 ). mRNAs or morpholinos were injected into the yolk of one-cell stage embryos, while plasmid DNAs or PCR-amplified DNAs were injected into the cytoplasm of one-cell stage embryos. When injected with a gfp -containing construct, embryos expressing GFP were picked up at desired stages and used for other manipulations. Injection doses were given in the corresponding figure legends. Whole-mount in situ hybridization and immunofluorescence Digoxigenin-labelled antisense RNA for each marker gene was in vitro synthesized. Whole-mount in situ hybridization was performed based on the standard procedures. Whole-mount immunofluorescence with a specific antibody was done along with DAPI staining and carried out essentially as before [63] , [64] . Equatorial or meridional cryostat sections of 8–10 μm were prepared following previously used procedures [65] ; only those sections that passed the organizer with a maximized plane as observed under a microscope were used for immunofluorescence. The section-containing slides were dried by heating at 65 °C in an oven for 4–8 h and then immunostained as for whole embryos. Immunostained embryos or sections were placed in an anti-fade reagent ( n -propyl gallate, 70% glycerol in PBS) and stored at −20 °C for up to 2 weeks. For successive in situ hybridization and immunofluorescence, embryos following in situ hybridization were subjected to immunofluorescence analysis. The used antibodies for immunofluorescence were as follows: rabbit anti-zebrafish Bmp2b(NT) antibody (Anaspec, 1:50 diluted), rabbit anti-zebrafish Chordin (GeneTex, 1:50 diluted), mouse anti-Smad1 antibody (Santa Cruz), rabbit anti-phospho-Smad1/5/8 (Cell Signaling, 1:100 diluted), mouse anti-β-catenin antibody (Cell signaling, 1:100 diluted), sheep anti-Digoxigenin antibody (Roche, 1:4,000 diluted), DyLight 488-conjugated AffiniPure Goat anti-mouse IgG and DyLight 549-conjugated AffiniPure goat anti-rabbit IgG secondary antibodies (Jackson ImmunoResearch, 1:100 diluted). Confocal imaging and signal measurement Immunostained embryos or sections were imaged under a Zeiss 710META or Nikon A1RMPSi lasers scanning confocal microscope. The whole-mount images were the sum of multiple focal planes (z-stack) using the software Image J or Bitplane-Imaris 7.6. Single focal plane images and the intensity of TRITC and DAPI in selected areas were analysed using NIS-Elements AR 4.1 software. For each selected area (323.28 μm 2 ), the ratio of TRITC/DAPI intensity was calculated and normalized. The average ratio was usually based on 3–5 sections or optical focal planes per embryo and a total of at least three embryos for each group. Luciferase reporter, western blot and ChIP assays Mammalian cell culture, transfection and luciferase reporter assays were done essentially as previously described [64] . Western blot using embryonic extracts at the 75% epiboly stage and luciferase assays in embryos at the shield stage also followed the previous protocols [64] . For ChIP assays, approximately 1,500 WT, MZoep or dorsomorphin-treated (1:1,000 for 6 h, Sigma) embryos were harvested at the shield stage for each assay and the procedures followed Liu et al . [66] using a mouse anti-Smad1 monoclonal antibody (Santa Cruz) that can recognize Smad1 and, to a lesser extent, Smad5. The primer sequences used for ChIP-PCR were: chd-f, 5′-CTCATCTGGTTCAATAGACAAG-3′; chd-r, 5′-TTCTGGAACTCTGACTGGA-3′; chd-ctr-f, 5′-GCTCTGCTGTCTTCACTC-3′; chd-ctr-r, 5′-GGTGGCGATGTTGATGAA-3′. The ChIP-PCR products were separated by gel electrophoresis, and the band intensity was analysed by using Image J software. Statistical analysis An average was expressed as mean±s.d. Significance of difference between two groups was analysed using Student’s t -test. Significant levels were indicated in corresponding context. Formulation of a mathematical model of Bmp and Chd gradients Ventrally synthesized Bmp, organizer Bmp or Chd, which are not bound by Chd or Bmp, are denoted by L , L′ or C , respectively. C binds to L at an on-rate k on creating the complex LC , and C binds to L ′ at an on-rate j on creating the complex L ′ C ; and the complexes LC and L ′ C are cleaved at the rates k off and j off , respectively. All components in our model, that is, L , L ′, C , LC and L ′ C , are allowed to diffuse with the respective diffusion coefficients D L , D L ′ , D C , D LC and D L ′ C , respectively. The concentrations of L , L ′ and C are denoted by [ L ], [ L ′] and [ C ], respectively, and the concentrations of LC and L ′ C are denoted by [ LC ] and [ L ′ C ], respectively. Then, the reaction-diffusion dynamics can be formulated as follows: where the parameters β L , β L ′ and β C are the degradation rates of L , L ′ and C , respectively; the parameters k deg and j deg are the degradation rates of the complexes LC and L ′ C , respectively; and the parameters V L , V L ′ and V C the synthesis rates of L , L ′ and C , respectively. In fact, the basic idea in mathematics behind this model is similar to the previous studies [14] , [39] , [40] . In our model, only one-dimensional geometry with length l is considered, where x =0 denotes the ventral extreme and x = l the dorsal extreme. The synthesis rates V L , V L ′ and V C in dynamics (1) are defined as where (i) S denotes the total level of the free Bmp ligands, that is, S =[ L ]+[ L ′]; (ii) and denote the possible maximum values of V L and V C , respectively; (iii) for V L ′ , the function δ( t ⩾ τ L ′ ) is defined as , that is, it represents that the synthesis of osBmp ( L′ ) will re-start at time t = τ L ′ and its synthesis rate is assumed to be a fixed constant for t ⩾ τ L ′ ; and (iv) the parameters T and T ′ are the fixed constants. In these definitions, V L is taken as a positive feedback function of total free Bmp level, that is, a Hill-type function of S with dV L / dS >0, and V C is taken to be a negative feedback function of total free Bmp level in the organizer, that is, also a Hill-type function of S but dV C / dS <0). Because a lower Bmp activity gradient led to chd expression in lateral and ventral margins outside the organizer ( Fig. 4j,k ), it is reasonable that a threshold is required for completely repressing chd expression. Therefore, for the synthesis of Chd on the x -axis with 0< x <11 l /12, we further assume that the synthesis rate of Chd at x is defined as where is a constant and the function is defined as , that is, when the local free Bmp level at x is lower (or higher) than a threshold level, denoted by s , the synthesis rate of Chd at this position is (or 0). The boundary and initial conditions of dynamics (1) are given below. Boundary conditions: All fluxes of diffusion components vanish at x =0 (ventral extreme) and at x = l (dorsal extreme), that is, the boundary condition can be expressed as for x =0 and x = l . Initial conditions: The initial values of the concentrations [ L ], [ L ′], [ C ], [ LC ] and [ L ′ C ], denoted by [ L ] 0 , [ L ′] 0 , [ C ] 0 , [ LC ] 0 and [ L ′ C ] 0 , respectively, are taken as for all possible 0≤ x ≤ l (refs 14 , 39 , 40 ). The setting values of the parameters in the numerical simulations were listed in Supplementary Table 1 , which were similar to those assumed by others [14] , [39] , [40] . How to cite this article: Xue, Y. et al . Organizer-derived Bmp2 is required for the formation of a correct Bmp activity gradient during embryonic development. Nat. Commun. 5:3766 doi: 10.1038/ncomms4766 (2014).